Achieving solar overall water splitting with hybrid photosystems of photosystem II and artificial photocatalysts Solar overall water splitting is a promising sustainable approach for solar-to-chemical energy conversion, which harnesses solar irradiation to oxidize water to oxygen and reduce the protons to hydrogen. The water oxidation step is vital but difficult to achieve through inorganic photocatalysis. However, nature offers an efficient light-driven water-oxidizing enzyme, photosystem II (PSII). Here we report an overall water splitting natural–artificial hybrid system, in which the plant PSII and inorganic photocatalysts (for example, Ru/SrTiO 3 :Rh), coupled with an inorganic electron shuttle [Fe(CN) 6 3− /Fe(CN) 6 4− ], are integrated and dispersed in aqueous solutions. The activity of this hybrid photosystem reaches to around 2,489 mol H 2 (mol PSII) −1 h −1 under visible light irradiation, and solar overall water splitting is also achieved under solar irradiation outdoors. The optical imaging shows that the hybrid photosystems are constructed through the self-assembly of PSII adhered onto the inorganic photocatalyst surface. Our work may provide a prototype of natural–artificial hybrids for developing autonomous solar water splitting system. Solar overall water splitting (OWS, 2 H 2 O→2 H 2 +O 2 ) to produce H 2 fuel is a promising approach for solar energy utilization [1] . Naturally, photosystem II (PSII), one of the photosynthetic enzymes responsible for the largest-scale solar-to-chemical energy conversion on earth, captures sunlight with wavelengths up to about 700 nm to drive water splitting into O 2 , protons and electrons using the Mn 4 CaO 5 cluster [2] , [3] , [4] . This primary process operates at nearly 100% quantum efficiency, and proceeds with a very small overpotential for water oxidation [5] . Therefore, from the viewpoint of using water as proton and electron sources for solar energy conversion, PSII is an extremely intriguing natural unit to be utilized for constructing hybrid systems, such as natural–artificial hybrid assembles between PSII and metal complexes/metal nanoparticles [6] , [7] , and PSII-based photo-bioelectrochemical device for generating photocurrent [8] , [9] , [10] . Although many efforts have been made on utilizing natural bioresources including PSII, photosystem I [11] , [12] , [13] and hydrogenase [14] , [15] to couple light energy conversion with water splitting, to our best knowledge, OWS reaction has not been realized by any reported natural–artificial hybrid systems. Artificially, numerous photocatalytic and photoelectrochemical systems have been constructed to provide a platform for generating photo-induced charge separation that is indispensable for proton reduction and/or water oxidation [16] , [17] , [18] , [19] . Nonetheless, only a limited number of artificial photosystems (mainly semiconductor-based photocatalysts) were found to be active by one-step photoexcitation for OWS [20] , [21] , [22] , while most of them are driven only by ultraviolet (UV) irradiation. Inspired by natural photosynthesis, two-step photoexcitation (that is, Z-scheme) has been proposed as an alternative approach to harness sunlight that mainly lies in visible and near infrared regions [17] . It has been recognized that the water oxidation (2 H 2 O→4 H + +4e − +O 2 ) half-reaction is the most challenging step for OWS in either the photocatalytic or photoelectrochemical process. While the hydrogen evolution (2 H + +2e − →H 2 ) half-reaction is relatively facile, as a result, many artificial inorganic photocatalysts have already shown high activity in this step [23] . However, it remains a long standing interest to realize OWS reaction by taking the advantages of natural PSII (oxygen evolution) and artificial photocatalyst (hydrogen production). Herein, we construct PSII–inorganic photocatalyst integrations ( Fig. 1 ) that can be well dispersed in aqueous solution. Two-step photoexcitation is employed in these natural–artificial hybrid photosystems, in which an inorganic donor/acceptor pair Fe(CN) 6 3 − /Fe(CN) 6 4 − acts as the electron shuttle from PSII to artificial photocatalysts. The electrochemical potential of this electron shuttle lies in between that of Q B (the terminal electron acceptor in PSII) and the valence band potential of semiconductor photocatalysts. Under visible light irradiation, this hybrid system shows the OWS activity up to 2,489 mol H 2 (mol PSII) −1 h − 1 , with H 2 /O 2 close to the stoichiometric ratio. This system also shows turnover number (based on PSII) of H 2 production as high as over 3,751. Interestingly, this system exhibits evident OWS activity without apparent loss of activity for at least over 3 h in direct sunlight. This work may inspire future developments of various solar-to-chemical energy approaches by taking the advantages of both natural photosynthesis and artificial photoelectrochemical processes. 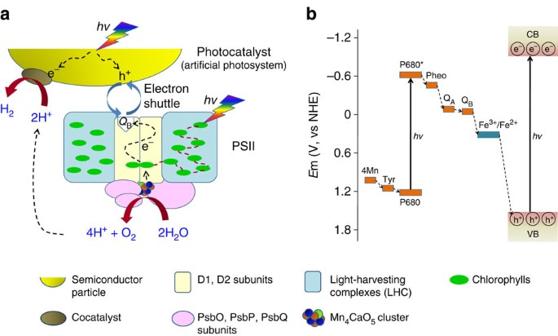Figure 1: Scheme of a PSII–photocatalyst hybrid system for OWS. (a) Illustrates the charge separation, electron flow and water splitting reaction in a PSII–photocatalyst hybrid system. (b) Indicates the band potential requirements of a semiconductor photocatalyst, for realizing the electron flow from PSII to photocatalyst, and proton reduction to H2. In PSII, light energy captured by light-harvesting complex (LHC) is rapidly funnelled into the chlorophylls bound in D1/D2 subunits, resulting in charge separation and a series of electron transfer finally toQBcofactor; O2evolution and proton (H+) release by water oxidation occurs on Mn4CaO5cluster. In photocatalyst, electrons generated by photoexcitation move to the surface and then relay on the cocatalyst for proton reduction into H2. Here, Fe3+/Fe2+redox cycle plays a role of electron shuttle betweenQBand h+(charged ‘hole’). The dash arrows denote the directions of electron, h+and proton transfers. For clarity, only D1, D2, PsbO, PsbP and PsbQ subunits of PSII are indicated ina. 4Mn, Tyr, P680, Pheo,QAandQBare the short names of the electron transfer cofactors in PSII; the conduction band and valence band of semiconductor photocatalysts are abbreviated as CB and VB, respectively. Figure 1: Scheme of a PSII–photocatalyst hybrid system for OWS. ( a ) Illustrates the charge separation, electron flow and water splitting reaction in a PSII–photocatalyst hybrid system. ( b ) Indicates the band potential requirements of a semiconductor photocatalyst, for realizing the electron flow from PSII to photocatalyst, and proton reduction to H 2 . In PSII, light energy captured by light-harvesting complex (LHC) is rapidly funnelled into the chlorophylls bound in D1/D2 subunits, resulting in charge separation and a series of electron transfer finally to Q B cofactor; O 2 evolution and proton (H + ) release by water oxidation occurs on Mn 4 CaO 5 cluster. In photocatalyst, electrons generated by photoexcitation move to the surface and then relay on the cocatalyst for proton reduction into H 2 . Here, Fe 3+ /Fe 2+ redox cycle plays a role of electron shuttle between Q B and h + (charged ‘hole’). The dash arrows denote the directions of electron, h + and proton transfers. For clarity, only D1, D2, PsbO, PsbP and PsbQ subunits of PSII are indicated in a . 4Mn, Tyr, P680, Pheo, Q A and Q B are the short names of the electron transfer cofactors in PSII; the conduction band and valence band of semiconductor photocatalysts are abbreviated as CB and VB, respectively. Full size image Isolated PSII membrane fragments The PSII membrane fragments, referred to as BBYs, were isolated from fresh spinach with non-ionic Triton X-100 detergent as described previously [24] . The polypeptide content was confirmed by SDS-polyacrylamide gel electrophoresis (see Supplementary Methods , Supplementary Fig. 1 ), indicating the three extrinsic polypeptides (PsbO, PsbP and PsbQ) remaining intact in the oxygen-evolving PSII samples. When the PSII sample (10 μg chlorophyll ml − 1 ) was suspended in a Na–phosphate buffer (pH 6.0), it was observed by microscopic imaging ( Fig. 2a ) that the green membrane fragments were inclined to stick together. 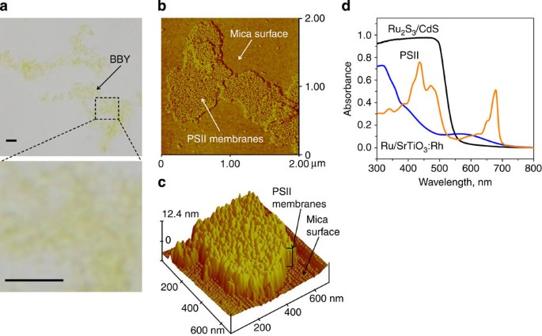Figure 2: Images of the PSII samples. (a) A bright-field microscope image of the PSII sample. (b) An AFM phase image of a piece of PSII membranes on a mica substrate. (c) Three-dimensional representation of an AFM height image from a piece of PSII membranes on a mica substrate. (d) UV-visible absorption spectra of PSII (orange), Ru2S3/CdS (black) and Ru/SrTiO3:Rh (blue). The spectra of these photocatalysts in powder form were measured with an integrating sphere for diffuse reflectance; this method is different from that using a cuvette for measuring the transmittance of the PSII solution; the results were finally transformed in absorbance. Fora,d, PSII of 10 μg chlorophyll ml−1was dispersed in a Na–phosphate buffer solution (50 mM sodium phosphates, 15 mM NaCl, pH 6.0). Scale bars, 5 μm. Figure 2: Images of the PSII samples. ( a ) A bright-field microscope image of the PSII sample. ( b ) An AFM phase image of a piece of PSII membranes on a mica substrate. ( c ) Three-dimensional representation of an AFM height image from a piece of PSII membranes on a mica substrate. ( d ) UV-visible absorption spectra of PSII (orange), Ru 2 S 3 /CdS (black) and Ru/SrTiO 3 :Rh (blue). The spectra of these photocatalysts in powder form were measured with an integrating sphere for diffuse reflectance; this method is different from that using a cuvette for measuring the transmittance of the PSII solution; the results were finally transformed in absorbance. For a , d , PSII of 10 μg chlorophyll ml − 1 was dispersed in a Na–phosphate buffer solution (50 mM sodium phosphates, 15 mM NaCl, pH 6.0). Scale bars, 5 μm. Full size image Atomic force microscopy (AFM) mapping of the isolated PSII membranes was performed to image the PSII arrangement in grana membrane. As shown in Fig. 2b,c , we observed a large number of PSII fragments on the mica surface. These two-dimensional AFM images and the three-dimensional representations ( Fig. 2b,c and Supplementary Fig. 2 ) are consistent with those reported by Helmut Kirchhoff et al . [25] for BBY sample under similar conditions. In Fig. 2b,c , the particles with protruding features represent the PSII enzyme embedded within the membrane [25] , [26] . Figure 2d (orange curve) shows the UV-visible absorption spectrum of the PSII sample. PSII is known to possess strong optical absorptions in the 400–520 and 600–700 nm ranges, with a weak-absorbing optical window region between 520 and 600 nm. These optical absorptions are originated from the pigments in PSII, and are dominated by the Soret ( λ max at 437 nm) and Q ( λ max at 679 nm) transitions of chlorophylls [27] and the π–π* transition ( λ max at 472 nm) of β-carotene [28] , [29] . H 2 -producing photocatalysts To construct the PSII–photocatalyst hybrid system for OWS, the bottom level of the conduction band of semiconductor-based photocatalyst must be more negative than the redox potential of H + /H 2 , while the top level of the valence band must be more positive than the midpoint potential of Q B / Q B − (around 0 V) [30] . In addition, for effective H 2 production, the photocatalyst should absorb light within the visible or infrared regions to complement those absorption bands from PSII. In this work, photocatalysts based on two typical semiconductors (CdS and SrTiO 3 :Rh (doped with Rh) powders) were adopted [17] . CdS, with a hexagonal structure (see Supplementary Methods ; Supplementary Fig. 3a ), was prepared through a hydrothermal method [31] . SrTiO 3 :Rh, with a Perovskite structure ( Supplementary Fig. 3b ), was synthesized by a solid-state reaction [32] . Ru 2 S 3 and Ru as cocatalysts were loaded on the surface of CdS and SrTiO 3 :Rh particles, respectively, by a photodeposition approach to improve photocatalytic activity [33] . Both Ru 2 S 3 /CdS and Ru/SrTiO 3 :Rh photocatalysts possess continuous optical absorptions down to visible region ( Fig. 2d ). In the ‘green’ region, which corresponds to the optical window for PSII, these photocatalysts possess, to some extent, complementary optical absorptions when compared with PSII. Both photocatalysts showed comparable activities in the photocatalytic proton reduction to H 2 when using Fe(CN) 6 4 − as the electron donor ( Supplementary Table 1 ). Self-assembly of the hybrid photosystems Here, we present a self-assembly approach to couple the PSII and photocatalyst under mild conditions. On the basis of the hydrophilic characteristic of the PSII membrane, the PSII membranes were expected to bind with the hydrophilic photocatalyst rather than the hydrophobic photocatalyst. Ru/SrTiO 3 :Rh is more hydrophilic (contact angle=28°) than Ru 2 S 3 /CdS (contact angle=90°), (see Supplementary Methods , Supplementary Fig. 4 ). The integration of PSII and photocatalyst was achieved in a Pyrex cell, which can be connected to a closed gas circulation and evacuation system for reaction test [31] ( Supplementary Fig. 5 ). Photocatalyst, electron mediator [Fe(CN) 6 3 − ] and PSII were sequentially dispersed in a Na–phosphate buffer at room temperature under stirring in the dark. The optical absorption spectrum of PSII-Ru 2 S 3 /CdS or PSII-Ru/SrTiO 3 :Rh aqueous mixture exhibits an overlapping broad background including both the characteristic absorptions of PSII (at 437, 472 and 679 nm) and the absorption band of CdS or SrTiO 3 :Rh semiconductor ( Supplementary Fig. 6 ). Correspondingly, these hybrid systems display deeper colour in comparison with the individual components ( Supplementary Fig. 7 ). 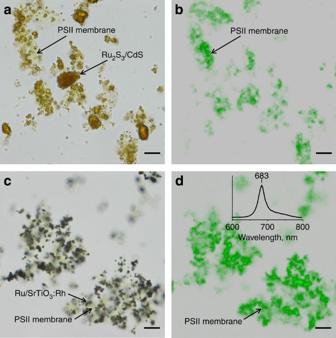Figure 3: Optical microscope images of the PSII–photocatalyst hybrid systems. (a,c) The bright-field microscope images of PSII-Ru2S3/CdS and PSII-Ru/SrTiO3:Rh hybrid systems, respectively. (b,d) The fluorescence intensity images of the exact same samples ina,c, respectively. This fluorescence signal originates from the chlorophylls bound in PSII, as illustrated by its spectrum in the inset ofd. Scale bars, 10 μm. Figure 3a,c shows the optical microscope images of PSII-Ru 2 S 3 /CdS and PSII-Ru/SrTiO 3 :Rh hybrid systems, respectively. For the PSII-Ru 2 S 3 /CdS system, it was found that a large portion of Ru 2 S 3 /CdS is self-aggregated into big particles (brown, around 10 μm in size), and the green PSII membranes as shown in Fig. 2a prefer to integrate with small Ru 2 S 3 /CdS particles rather than the big aggregates. For PSII-Ru/SrTiO 3 :Rh system ( Fig. 3c and Supplementary Fig. 8 ), the green PSII membranes clearly bind to the dark Ru/SrTiO 3 :Rh particles, and these hybrid integrations are well dispersed in the aqueous buffer ( Supplementary Figs 7 and 8 ). These integrations of PSII and photocatalysts (Ru 2 S 3 /CdS, Ru/SrTiO 3 :Rh) are also illustrated by the fluorescence images of the chlorophylls that bound in PSII ( Fig. 3b,d ). Note that no such transient fluorescence signal can be detected from Triton X-100 detergent, Ru 2 S 3 /CdS, or Ru/SrTiO 3 :Rh under these conditions. When placing Fig. 3b over Fig. 3a , or Fig. 3d over Fig. 3c , we can see that the fluorescence images exactly overlap the bright field images of the PSII membranes, adhering to those photocatalyst particles. Figure 3: Optical microscope images of the PSII–photocatalyst hybrid systems. ( a , c ) The bright-field microscope images of PSII-Ru 2 S 3 /CdS and PSII-Ru/SrTiO 3 :Rh hybrid systems, respectively. ( b , d ) The fluorescence intensity images of the exact same samples in a , c , respectively. This fluorescence signal originates from the chlorophylls bound in PSII, as illustrated by its spectrum in the inset of d . Scale bars, 10 μm. Full size image OWS of the hybrid photosystems OWS reactions of the hybrid systems were performed under visible light irradiation ( λ >420 nm, with a xenon lamp). Simultaneous evolutions of H 2 and O 2 were detected ( Fig. 4a,c,d ). For PSII-Ru 2 S 3 /CdS, at pH 6.0, the OWS activity reaches to around 411 mol H 2 (mol PSII) − 1 h − 1 with the molar ratio H 2 :O 2 close to 2:1 after 1 h irradiation, indicating the stoichiometric production of H 2 and O 2 directly from OWS. When the photocatalyst, Ru 2 S 3 /CdS was replaced with Ru/SrTiO 3 :Rh, the activity was significantly increased up to around 2,489 mol H 2 (mol PSII) − 1 h − 1 and 1,334 mol O 2 (mol PSII) − 1 h − 1 in the first hour. Importantly, this oxygen evolution rate is close to that of the half-reaction using PSII alone under the same conditions ( Supplementary Fig. 9 and Table 1 ). This result supports that the presence of the inorganic photocatalyst in the hybrid system does not significantly affect the integrity of the PSII. In addition, the turnover number (based on PSII) is estimated to be over 3,751 in 2 h ( Fig. 4c ), suggesting that the PSII in the hybrid system is stable. At pH 7.0, the OWS activities drop severely for both hybrid systems. This phenomenon is well associated with the O 2 evolution behaviour of PSII alone at different pH values ( Supplementary Fig. 10 and Table 1 ). 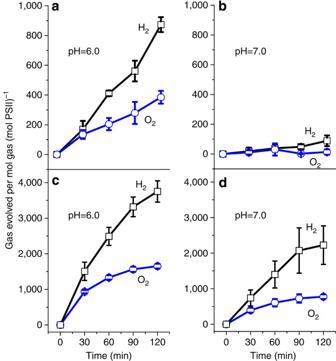Figure 4: Time courses of OWS by the PSII–photocatalyst hybrid systems. (a,b) OWS by PSII-Ru2S3/CdS at pH 6.0 and 7.0, respectively. (c,d) OWS by PSII-Ru/SrTiO3:Rh at pH 6.0 and 7.0, respectively. The light source was a xenon lamp with a long-pass filter (λ>420 nm) and the power density was 250 mW cm−2. All data points represent the average of three independent data sets with s.d. Figure 4: Time courses of OWS by the PSII–photocatalyst hybrid systems. ( a , b ) OWS by PSII-Ru 2 S 3 /CdS at pH 6.0 and 7.0, respectively. ( c , d ) OWS by PSII-Ru/SrTiO 3 :Rh at pH 6.0 and 7.0, respectively. The light source was a xenon lamp with a long-pass filter ( λ >420 nm) and the power density was 250 mW cm −2 . All data points represent the average of three independent data sets with s.d. Full size image Table 1 Visible light-driven water-splitting activities of the hybrid systems. Full size table The fact that only O 2 evolution was detected ( Fig. 5 ) for both hybrid systems under red light irradiation ( λ >600 nm, out of the optical absorption ranges of the photocatalysts) unambiguously confirms that the artificial components (Ru 2 S 3 /CdS, Ru/SrTiO 3 :Rh) of the hybrid systems are indispensible for OWS. In addition, it was found that the oxygen evolution activity of the PSII-Ru/SrTiO 3 :Rh hybrid was much higher than that of PSII-Ru 2 S 3 /CdS hybrid under red light irradiation. This result suggests that an interaction between PSII and Ru 2 S 3 /CdS might result in conformational changes to the PSII enzyme, thus decreasing oxygen evolution efficiency. 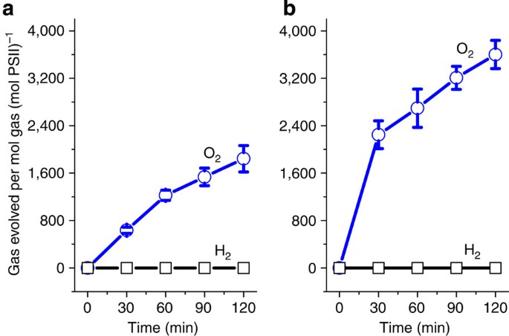Figure 5: Time courses of red light-driven water splitting by the hybrid systems. (a) PSII-Ru2S3/CdS. (b) PSII-Ru/SrTiO3:Rh. Both hybrid systems were dispersed in the Na–phosphate buffer solution with pH 6.0. The light source was a xenon lamp with a long-pass filter (λ>600 nm) and the power density was 150 mW cm−2. All data points represent the average of three independent data sets with s.d. Figure 5: Time courses of red light-driven water splitting by the hybrid systems. ( a ) PSII-Ru 2 S 3 /CdS. ( b ) PSII-Ru/SrTiO 3 :Rh. Both hybrid systems were dispersed in the Na–phosphate buffer solution with pH 6.0. The light source was a xenon lamp with a long-pass filter ( λ >600 nm) and the power density was 150 mW cm − 2 . All data points represent the average of three independent data sets with s.d. Full size image Interestingly, OWS by the PSII-Ru/SrTiO 3 :Rh hybrid was also conducted under direct sunlight outdoors ( Supplementary Fig. 11 ). As shown in Fig. 6 , H 2 and O 2 simultaneously evolve, and solar OWS activity remains during a 3-h test. 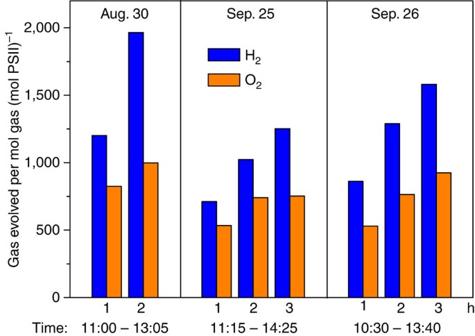Figure 6: Time courses of solar OWS by PSII-Ru/SrTiO3:Rh. This hybrid system was dispersed in the Na–phosphate buffer solution with pH 6.0. The light source was sunlight in Dalian city in 2013. Figure 6: Time courses of solar OWS by PSII-Ru/SrTiO 3 :Rh. This hybrid system was dispersed in the Na–phosphate buffer solution with pH 6.0. The light source was sunlight in Dalian city in 2013. Full size image To verify in the hybrid systems that the electrons, used for H 2 production, originate from the water oxidation (2H 2 O→O 2 +4e − +4H + ) by PSII, hybrid systems containing Mn-depleted PSII were constructed and tested for the OWS reaction. In the case of Mn-depleted PSII, in which Mn 4 CaO 5 cluster as well as PsbO, PsbP and PsbQ extrinsic polypeptides were removed by Tris treatment ( Supplementary Fig. 1 ), no O 2 evolution was detected in the water splitting testing and only a small amount of H 2 was detected due to the background reactions of the photocatalysts ( Table 1 and Supplementary Table 1 ). A similar result was obtained for the hybrid systems ( Table 1 ) when 3-(3,4-dichlorophenyl)-1,1-dimethylurea, a well-known inhibitor for terminating the electron transfer of PSII by occupying Q B site, was added. Therefore, these control experiments unambiguously demonstrate that the electrons supplied from water oxidation in PSII are transferred to the artificial inorganic photocatalyst, which utilizes the electrons to couple with protons to generate H 2 . In summation, the OWS takes place within the natural–artificial hybrid systems, PSII-Ru 2 S 3 /CdS or PSII-Ru/SrTiO 3 :Rh, under visible light irradiation, and O 2 evolution from the water-oxidizing PSII enzyme supplies electrons and protons, which in turn are employed by the inorganic photocatalysts to produce H 2 . In this work, hybrid photosystems with PSII and artificial photocatalysts have been constructed for autonomous visible light-driven OWS. To transport the electrons from PSII to the photocatalysts, the Fe(CN) 6 3 − /Fe(CN) 6 4 − ( E o =0.358 V versus NHE) [34] redox cycle was employed as the electron shuttle, because its electrochemical potential lies between that of PSII cofactor Q B (around 0 V) [30] and the top level (1.5 V) [33] of the valence band potential of CdS and the level (2.2 V) [32] of Rh 3+ doped in SrTiO 3 :Rh. On accepting an electron from PSII, Fe(CN) 6 3 − is reduced to Fe(CN) 6 4 − ( Supplementary Fig. 12 ) [35] , which returns to Fe(CN) 6 3 − after donating an electron to the photocatalyst. Electron donation was confirmed with the half-reaction test for the photocatalytic hydrogen production by the inorganic photocatalyst ( Supplementary Fig. 13 and Supplementary Table 1 ). The OWS activity of PSII-Ru/SrTiO 3 :Rh hybrid system was found to be dependent on the initial concentration of the electron mediator, Fe(CN) 6 3 − ( Supplementary Fig. 14 ). This correlates well with the oxygen evolution of isolated PSII using Fe(CN) 6 3 − as exogenous electron acceptor as shown in Supplementary Fig. 12 , in which the trace can be well explained by the Michaelis–Menten equation. Therefore, these results lead us to the conclusion that the transportation of electron from PSII is the rate-limiting process for this hybrid system. For these hybrid photosystems, the overall efficiency of light energy conversion ( η ) for proton reduction to generating H 2 by the inorganic photocatalyst is much higher than that for water oxidation to generating O 2 by the PSII (see Supplementary Table 1 ). For instance, η of Ru/SrTiO 3 :Rh is over three times η of PSII when 5 mM electron mediator is used. This is likely the main reason why the molar ratio H 2 :O 2 for water splitting by the hybrid photosystem is close to 2:1 when only ferricyanide is added, in which case the generated ferrocyanide is estimated to be much less. It was also noted that the isolated PSII membranes were damaged when illuminated for a few hours ( Supplementary Fig. 9 ). The stability of these hybrid photosystems under illumination seems to be dependent on that of their component PSII, because the inorganic photocatalysts are much stable during the photocatalytic reactions for hours [31] , [32] . The PSII damage can be partly due to the effects of photo-oxidative stress on the protein structure. As side reactions, the triplet chlorophyll formed in the antenna and reaction centre of PSII complexes can convert ground state O 2 into highly reactive singlet oxygen, 1 O 2 (refs 36 , 37 ). Other types of reactive oxygen species (ROS), such as O 2 • − , H 2 O 2 and HO • , could be produced on the reducing side or oxidizing side of PSII [38] . Although the amounts of the generated ROS are limited, it has been demonstrated that exposure of isolated PSII complexes to ROS, such as 1 O 2 or H 2 O 2 , results in specific cleavage of the core polypeptide, D1 (refs 39 , 40 ). Other origins of causing PSII inactivation are probably associated with the disruption of the oxygen-evolving complex with the release of manganese ions by excess blue light irradiation [41] , and the photodamage occurring at the reaction centre with excited chlorophyll [41] , [42] . By investigating the influence of illumination with different wavelength ranges on the activity and stability of the isolated PSII membranes, the illumination with λ >600 nm was shown to be more positive compared with the illumination with λ >420 nm ( Supplementary Fig. 9 ). For the hybrid photosystems, the component Ru 2 S 3 /CdS or Ru/SrTiO 3 :Rh photocatalyst possesses continuous optical absorption above 420 nm ( Fig. 2d ). Therefore, the light absorption of the photocatalysts could, to some extent, alleviate the photodamage of PSII in the hybrid photosystems. Through a self-assembly approach, the PSII membrane fragments can be easily bound to the surface of Ru/SrTiO 3 :Rh particles via hydrophilic interactions, forming well-distributed hybrid integration. In comparison with PSII-Ru/SrTiO 3 :Rh (contact angle=28°, Supplementary Fig. 4a ), the PSII membranes are not uniformly binding to the Ru 2 S 3 /CdS (contact angle=90°, Supplementary Fig. 4b ) particles ( Fig. 3 ). This probably results from the hydrophobic characteristic of the Ru 2 S 3 /CdS surface and may be one of the reasons for the relatively lower OWS activity of the PSII-Ru 2 S 3 /CdS hybrid system ( Fig. 4 ). The present work has demonstrated a bioartificial hybrid photosystem that is self-assembled via the interaction between the PSII membrane and the surface of semiconductor-based photocatalyst. The hybrid system dispersed in the aqueous solution can split water into H 2 and O 2 without any sacrificial reagent under visible light irradiation. The electrons from water oxidation by PSII are shuttled to the Ru/SrTiO 3 :Rh or Ru 2 S 3 /CdS photocatalyst for proton reduction via a Fe(CN) 6 3 − /Fe(CN) 6 4– electron mediator. Interestingly, the resulting activities of OWS between the PSII-Ru/SrTiO 3 :Rh hybrid (around 2,489 mol H 2 (mol PSII) − 1 h − 1 ) and the PSII-Ru 2 S 3 /CdS hybrid (around 411 mol H 2 (mol PSII) − 1 h − 1 ) are quite different, probably due to the interaction of PSII protein with the surface of inorganic materials with different hydrophilic property, which may lead to conformation changes of the subunit proteins of PSII enzyme complex. Our work provides a prototype of natural–artificial hybrid for developing autonomous solar OWS system. Preparation of the PSII samples The PSII membrane fragments (called as BBY) were isolated from fresh spinach as described previously [24] . These PSII samples (~2 mg chlorophyll ml − 1 ) were finally suspended in a SMN buffer (400 mM sucrose, 50 mM MES-NaOH, 15 mM NaC1, pH 6.0), and then frozen in liquid nitrogen and stored at −70 °C. The O 2 evolution activities of these PSII samples are over 800 μmol O 2 (mg of chlorophyll) − 1 h − 1 measured in the SMN buffer, and around 750 μmol O 2 (mg of chlorophyll) − 1 h − 1 in a Na–phosphate buffer (pH 6.0) with a Clark-type oxygen electrode at 25 °C. The total chlorophyll concentrations of the PSII samples were determined according to the following equation, which is based on the optical absorption coefficients of chlorophyll a and b in an 80% acetone aqueous solution [43] . A is the measured absorbance at the indicated wavelength. The concentrations of the PSII reaction centre (RC) were calculated according to [Chl]/[RC]=274, which was previously determined by reverse-phase high-performance liquid chromatography [44] . To qualify these PSII samples, the steady-state O 2 evolution of these PSII samples at 25 °C under saturated red light illumination was monitored with a Clark-type oxygen electrode [45] . The PSII sample corresponding to 40 μg chlorophyll, 0.53 mM recrystallized 2,6-dichlorobenzoquinone and 1 mM potassium ferricyanide were dispersed in a buffer. The total assay volume was 3.0 ml. The O 2 evolution rate was estimated from the O 2 concentration change during the initial 20 s on illumination. Air-saturated water was used as an oxygen standard. For the preparation of the Mn-depleted PSII, the Mn 4 CaO 5 cluster as well as PsbO, PsbP and PsbQ polypeptides were removed from BBY by Tris treatment with a buffer (pH 8.0) containing 0.8 M tris(hydroxymethyl)-aminomethane (Tris) and 2.0 mM EDTA (ethylenediaminetetraacetic acid), as described previously [46] . These Mn-depleted PSII samples (~2 mg chlorophyll ml − 1 ) were finally suspended in a SMN buffer (400 mM sucrose, 50 mM MES-NaOH, 15 mM NaC1, pH 6.0), and then frozen in liquid nitrogen and stored at −70 °C. The O 2 evolution activities of these Mn-depleted PSII samples are too low to determine. But, these samples remained good capability of light-induced electron transfer when exogenous electron donor (1,5-diphenylcarbazide) and acceptor (2,6-dichloroindophenol sodium salt) were added. Preparation of the photocatalysts The CdS powder was prepared by the same method as employed in a previous study [31] . Eight hundred millilitres of 0.14 M Na 2 S aqueous solution was added slowly to 1,000 ml of 0.14 M Cd(OAc) 2 aqueous solution under vigorous stirring. This yellow mixture was stirred for 24 h and kept for additional 24 h. The slurry was collected by filtration and transferred into a teflon-lined stainless steel autoclave, and then heated at 200 °C for 72 h. The formed powder was filtered, and washed subsequently with water and ethanol before drying. The cocatalyst Ru 2 S 3 (0.2 wt%) was loaded on CdS (denote as Ru 2 S 3 /CdS) by photodeposition. Briefly, a RuCl 3 aqueous solution was added dropwise to a suspension of CdS powder (0.5 g) in 0.5 M Na 2 S aqueous solution. This mixture was degassed under vacuum and then irradiated for 30 min. The obtained Ru 2 S 3 /CdS particles was centrifuged, washed with water and finally dried at 50 °C under vacuum. The SrTiO 3 :Rh (SrTiO 3 doped with Rh) powder was synthesized by a solid-state reaction [32] . SrCO 3 , TiO 2 and Rh 2 O 3 were mixed evenly in a mortar according to the molar ratio Sr:Ti:Rh=1.03:1:0.01. This mixture was calcined at 1,100 °C for 10 h. The cocatalyst Ru (0.5 wt%) was loaded on SrTiO 3 :Rh (denote as Ru/SrTiO 3 :Rh) by photodeposition as reported previously [47] . Briefly, a RuCl 3 aqueous solution was added dropwise to a suspension of SrTiO 3 :Rh powder (0.5 g) in a 10% methanol aqueous solution. This mixture was degassed under vacuum and then irradiated for 6 h. The obtained Ru/SrTiO 3 :Rh particles was filtered, washed with water and finally dried at 50 °C under vacuum. Preparation of the PSII–photocatalyst hybrid systems Photocatalyst powder (0.1 g) was first dispersed in 100 ml of the buffer solution (50 mM sodium phosphates, 15 mM NaCl, pH 6.0 or pH 7.0) by sonication. Next, potassium ferricyanide (Fe(CN) 6 3 − , 5 mM) was dissolved in this solution, and then the PSII (1 mg chlorophyll) previously thawed on ice in the dark was added slowly under stirring at room temperature in the dark. Once the assembly was completed, this aqueous mixture would be used for water splitting test. For the control experiments ( Table 1 ), the oxygen-evolving PSII was replaced by the same amount of Mn-depleted PSII, in which Mn 4 CaO 5 cluster as well as PsbO, PsbP and PsbQ extrinsic polypeptides were removed; or, 3-(3,4-dichlorophenyl)-1,1-dimethylurea (12 μM) was added to the PSII solution under stirring for 2 min in the dark, before mixed with the photocatalysts. OWS reaction For water splitting tests of the PSII–photocatalyst hybrid integrations, the aqueous mixture (PSII–photocatalyst integrations, Fe(CN) 6 3 − , sodium phosphates, NaCl) was transferred to a reaction test system ( Supplementary Fig. 5 ), where this aqueous mixture was thoroughly degassed under vacuum and maintained at 25 °C. The visible light-driven water splitting reaction was conducted by the irradiation (250 mW cm − 2 ) from a xenon lamp with a long-pass filter ( λ >420 nm). The amounts of H 2 and O 2 evolution were monitored by online gas chromatography (5A zeolite column and Ar carrier gas, Agilent GC 7890, USA). The water splitting tests of other reactant combinations were performed in a similar way, unless specific mentions. Sunlight-driven water splitting reaction The PSII-Ru/SrTiO 3 :Rh hybrid system, which was constructed by self-assembly of Ru/SrTiO 3 :Rh (0.1 g ), PSII (1 mg chlorophyll) and Fe(CN) 6 3 − (8.4 mM) in 60 ml of the buffer solution (50 mM sodium phosphates, 15 mM NaCl, pH 6.0) sealed in a flask, was degassed thoroughly under vacuum and then filled with Ar gas. This flask filled with the aqueous mixture was immerged into a big beaker of water, which can filter the infrared of sunlight. This whole setup ( Supplementary Fig. 11 ) was exposed outdoors for sunlight-driven water splitting test. Samples (200 μl of gas) were taken from the headspace in the flask every hour, and analysed by gas chromatography to determine H 2 and O 2 evolutions. During the reaction, the aqueous mixture was under stirring, and cold water was added to the beaker to maintain ~25 °C. The light source was sunlight in Dalian city in 2013. The irradiation area for reaction test was ~26 cm 2 . AFM Samples were prepared by placing a 20-μl drop of PSII solution (10 μg chlorophyll ml − 1 ) on a freshly cleaved mica surface (8 × 13 mm) for 10 min, and washed with water for five times to remove the buffer. The retained water was then removed from the mica surface with an air stream. AFM imaging was carried out in a tapping mode in air (Nanoscope 3D, Veeco, USA). Antimony-doped silicon cantilevers (tip radii of 8 nm) with resonant frequencies of 280–350 kHz were used and nominal spring constant was 20 N/m. UV-visible absorption spectroscopy The UV-visible absorption spectra of the PSII samples were recorded on a spectrophotometer (Cary 50, VARIAN, USA). PSII (10 μg chlorophyll ml − 1 ) was diluted in the buffer solution (50 mM sodium phosphates, 15 mM NaCl, pH 6.0), which was also used as the reference for spectral measurement. The parameters were: band width, 1.5 nm and scan speed, 600 nm min −1 . The UV-visible absorption spectra of the photocatalyts were recorded on a spectrophotometer (V-550, JASCO, Japan), which includes an integrating sphere for diffuse reflectance. The Kubelka–Munk theory was adopted to portray the reflectance data with BaSO 4 as the reference. The parameters were: band width, 2.0 nm and scan speed, 400 nm min −1 . Optical imaging and fluorescence spectroscopy These characterizations were implemented by a combined instrument, which consists of a microscope (IX81, Olympus, Japan), a laser confocal scanning fluorescence lifetime imaging microscopy system (LCS-FLIM; DCS120, B&H, Germany) and a home-built spectrometer. Aqueous samples at room temperature were held between the microscope slide and coverslip without any treatment. For fluorescence measurements, a laser (405 nm in wavelength, ~200 nW in power) was used as excitation source. By the time-correlated single photon counting approach, the transient fluorescence signal in the range 600–900 nm was collected as data source for the fluorescence intensity imaging of the samples. The scan settings were: 5 μs per pixel, 0.414 s per frame and 49 frames in total. The fluorescence spectra were recorded on an intensified charge-coupled device detector, which coupled with a monochromator. How to cite this article: Wang, W. et al . Achieving solar overall water splitting with hybrid photosystems of photosystem II and artificial photocatalysts. Nat. Commun. 5:4647 doi: 10.1038/ncomms5647 (2014).